In situmeasurement of exciton energy in hybrid singlet-fission solar cells Singlet exciton fission-sensitized solar cells have the potential to exceed the Shockley–Queisser limit by generating additional photocurrent from high-energy photons. Pentacene is an organic semiconductor that undergoes efficient singlet fission—the conversion of singlet excitons into pairs of triplets. However, the pentacene triplet is non-emissive, and uncertainty regarding its energy has hindered device design. Here we present an in situ measurement of the pentacene triplet energy by fabricating a series of bilayer solar cells with infrared-absorbing nanocrystals of varying bandgaps. We show that the pentacene triplet energy is at least 0.85 eV and at most 1.00 eV in operating devices. Our devices generate photocurrent from triplets, and achieve external quantum efficiencies up to 80%, and power conversion efficiencies of 4.7%. This establishes the general use of nanocrystal size series to measure the energy of non-emissive excited states, and suggests that fission-sensitized solar cells are a favourable candidate for third-generation photovoltaics. Of the options for renewable energy, photovoltaic technologies [1] , [2] , [3] with the potential to exceed the Shockley–Queisser limit [4] on single bandgap devices are particularly attractive [5] , [6] , [7] , [8] . One strategy is to sensitize a low-bandgap semiconductor with a higher bandgap material that can generate additional photocurrent from absorbed high-energy photons [6] , [9] . Such an opportunity is offered by singlet fission, which is the spin-conserving process by which a spin-singlet exciton on an organic chromophore splits to form a pair of lower-energy triplet excitons on neighbouring molecules [10] . Transient optical absorption measurements suggest that this process can be highly efficient, as we have observed singlet fission occurring on an 80 fs timescale in pentacene [11] . The significance of singlet exciton fission for solar cells is that, if both triplets can be ionized, it possibly permits performance above the Shockley–Queisser limit on power conversion efficiency [4] without requiring a current-matched tandem photovoltaic device [9] . However, this potential has not been realized to date [3] . Pentacene is an attractive material for a sensitizer as it undergoes efficient singlet fission [11] , [12] , [13] and has high hole mobility [14] , but the triplet energy is challenging to determine because of the vanishingly small photoluminescence quantum yield of pentacene [10] , [15] . In the solid state the triplet energy has been measured indirectly using variable-temperature host-guest fluorescence [16] , electron backscattering from crystalline pentacene [17] , and inelastic tunnelling spectroscopy on amorphous pentacene [18] . In solution it has been studied using broadband flash photolysis [19] , [20] , [21] , and estimated via a range of theoretical calculations [22] , [23] , [24] , [25] , [26] . However it is unclear that these energies are relevant to ionization at a polycrystalline pentacene heterojunction. More broadly, it would be beneficial to examine the energy of non-emissive states [27] under photovoltaic operating conditions [28] , but a tunable probe of this kind is lacking. We have previously demonstrated that pentacene can be used in a fission-sensitized photovoltaic device with inorganic nanocrystals as the infrared absorbers [29] . Colloidal nanocrystals have generated broad interest for use in photovoltaic devices [30] , [31] . Alivisatos and co-workers used nanocrystals in photovoltaics dispersed in polymer matrices [32] , and subsequent studies have investigated bilayer structures [33] and hybrid organic/inorganic junctions [34] . There has also been steady progress in lead chalcogenide nanocrystal solar cells in a variety of device architectures [5] , [6] , [7] , [35] , [36] . In spite of this progress, there is a broad recognition of the need for innovations in materials. For instance, a narrower nanocrystal size distribution is expected to yield better performance owing to a greater uniformity of percolation networks [37] and a decrease in interstitial volume [38] . The tunable energy states of colloidal nanocrystals also make them well suited to probe solar cell device energetics. For semiconductor nanocrystals smaller than the radius of the Bohr exciton, the nanocrystal surface boundary imposes a confining potential on the electrons and holes that varies with the nanocrystal size. Hence, the ability to synthesize nanocrystals of different sizes leads to materials with different state energies. Additionally, when the nanocrystal size series is composed of the same inorganic semiconductor and organic ligands, the state tunability (including the energy of the lowest energy absorption) is largely decoupled from the bulk dielectric and chemical properties of the materials [39] , [40] . Thus, by incorporating nanocrystals with different sizes and hence different state energies into working devices, it is possible to assess energetic parameters of device performance. The precision of a size series experiment for nanocrystal devices depends on both the degree of monodispersity within a particular nanocrystal sample and the ability to access a range of distinct nanocrystal sizes. Previously, our group fabricated photovoltaic devices with pentacene/lead sulphide (PbS) nanocrystal heterojunctions [29] . However, PbS nanocrystal syntheses often yield only moderately monodisperse samples, presumably owing to the rapid reaction of their precursors [41] , [42] , [43] . In this study, we fabricate bilayer photovoltaic cells with pentacene, using lead selenide (PbSe) nanocrystals as the infrared absorbing material. In contrast to PbS, the syntheses of PbSe nanocrystals yield samples with greater monodispersity, making them suitable as probes of operation energies in devices. Although the bulk PbSe bandgap is smaller than that of PbS, there is a greater degree of confinement for PbSe and hence the size-dependent energy levels of PbS and PbSe cover a range that is well-matched to pentacene [44] . PbSe nanocrystals The absorption spectra of our PbSe nanocrystal size series are shown in Fig. 1 , and the lowest-energy absorption maxima of the nanocrystals (1S e –1S h ) range from 0.67 to 1.3 eV in solution. Although we synthesized nanocrystals using two different hot injection methods, every sample in the size series was prepared using identical precursors to ensure all surfaces would be directly comparable. The nanocrystal samples have polydispersities of 3–6%. 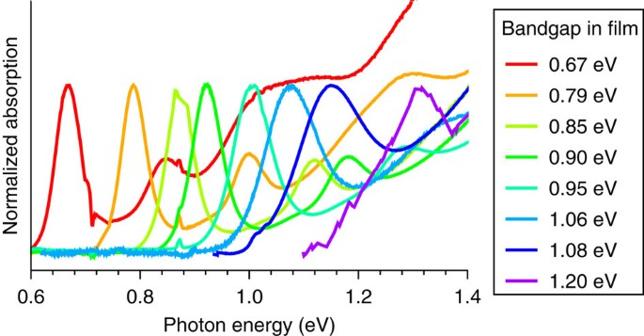Figure 1: PbSe nanocrystal absorption spectra. Absorption spectra of the lead selenide (PbSe) semiconductor nanocrystals used during this study, in solution. The nanocrystals range in monodispersity from 3–6%. Curves are labelled with the nanocrystal bandgap in the film. Figure 1: PbSe nanocrystal absorption spectra. Absorption spectra of the lead selenide (PbSe) semiconductor nanocrystals used during this study, in solution. The nanocrystals range in monodispersity from 3–6%. Curves are labelled with the nanocrystal bandgap in the film. Full size image To determine the energies of the lowest-lying nanocrystal states with respect to vacuum, we investigated PbSe nanocrystal films formed on pentacene via ultraviolet photoelectron spectroscopy (UPS) (see Supplementary Fig. S1 and Supplementary Table S1 ). The onset of the lowest-energy ionization feature at −5.1 eV varies by only 0.03 eV over the nanocrystal size series (within the measurement error of 0.05 eV) even though the optical gap set by the lowest absorption varies by 0.6 eV. This indicates that quantum confinement affects the conduction band state (1S e ) much more strongly than the valence band state (1S h ) [44] . We also found that the energy of the highest occupied molecular orbital in pentacene is −5.05±0.05 eV, in accordance with earlier measurements [45] , [46] . Triplet energy determination To study the energy states of pentacene that are relevant to singlet fission, our photovoltaic devices were fabricated as follows. The pentacene and PbSe active layers were deposited in a bilayer structure on indium-tin oxide (ITO), such that incident light first passes through pentacene to absorb higher-energy photons. PbSe nanocrystals were spun-cast on top of the sublimed pentacene via a layer-by-layer technique. The top contacts consist of a thin layer of lithium fluoride and an aluminium electrode. To highlight the pentacene contribution, we used devices that had a nanocrystal layer thickness of 50 nm and benefit from the favourable photonic structure imposed by the reflective aluminium electrode [29] . The device structure is illustrated in Fig. 2 . 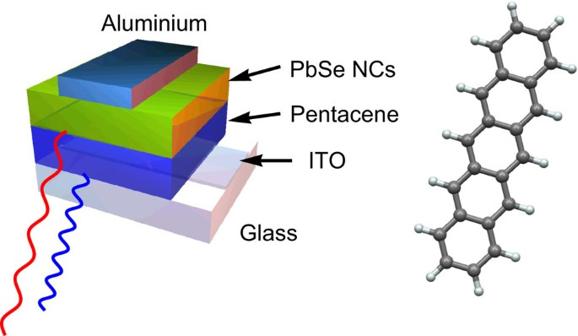Figure 2: Photovoltaic device structure. Schematic of the devices used in this study and chemical structure of pentacene. Pentacene was evaporated on ITO-coated glass substrates. PbSe nanocrystals were spin-coated on top of pentacene, followed by thermal evaporation of aluminium. A lithium fluoride layer was present between the aluminium and the nanocrystals in the devices optimized for power conversion efficiency. Figure 2: Photovoltaic device structure. Schematic of the devices used in this study and chemical structure of pentacene. Pentacene was evaporated on ITO-coated glass substrates. PbSe nanocrystals were spin-coated on top of pentacene, followed by thermal evaporation of aluminium. A lithium fluoride layer was present between the aluminium and the nanocrystals in the devices optimized for power conversion efficiency. Full size image The spectral dependence of the short-circuit photocurrents (external quantum efficiency (EQE) spectra) for the series of photovoltaic devices are shown in Fig. 3 and Supplementary Fig. 2 . The onset of photocurrent ( Supplementary Fig. S3 ) corresponds to the absorption onset of nanocrystals in the film, which occurs at a lower energy than the absorption of the same nanocrystals in solution ( Supplementary Fig. S4 ). For the purposes of this discussion and in accordance with UPS analysis, we identify the photocurrent onset determined from EQE spectra ( Supplementary Fig. S5 ) as the relevant bandgap energy of the nanocrystals ( E PCO ). 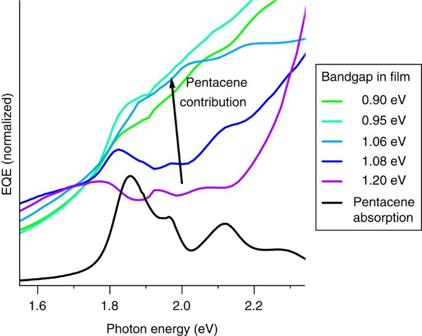Figure 3: Pentacene contribution in nanocrystal/pentacene solar cells. Normalized external quantum efficiency spectra of pentacene photovoltaic devices prepared with a size series of PbSe. We observe a contribution from pentacene in devices with nanocrystals up to 1.08 eV, indicated with an arrow. Figure 3: Pentacene contribution in nanocrystal/pentacene solar cells. Normalized external quantum efficiency spectra of pentacene photovoltaic devices prepared with a size series of PbSe. We observe a contribution from pentacene in devices with nanocrystals up to 1.08 eV, indicated with an arrow. Full size image Current-voltage characteristics of photovoltaic devices ( Supplementary Fig. S6 ) demonstrate that devices with nanocrystals of all bandgaps exhibit qualitatively similar device behaviour. From the UPS results, we expect changes in PbSe nanocrystal confinement to affect predominantly the 1S e energy. This result is consistent with the strong correlation between the nanocrystal bandgap ( E PCO ) and the open-circuit voltage ( V oc , Fig. 4 ), with a slope close to unity. The axis intercept of only 0.42 V indicates a voltage loss close to the lowest achievable limit [47] . Additionally, the high EQE maxima indicate that charge carriers in the nanocrystals are separated efficiently. This result shows that even the small (0.05 eV) difference between the smallest-gap nanocrystal 1S h energy and the pentacene HOMO is sufficient for hole transfer across the nanocrystal/pentacene interface. As this energy difference is equal to the error of our UPS measurements, we conclude that the energy required for hole transfer across the nanocrystal/pentacene heterojunction is small. 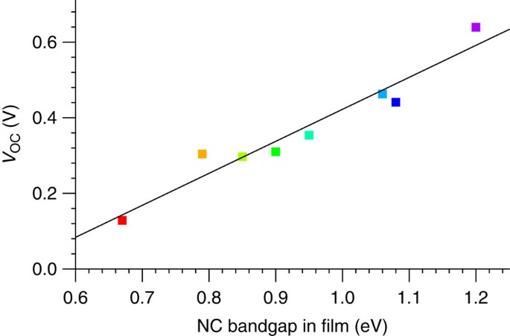Figure 4:Vocvariation with nanocrystal bandgap. Variation of open-circuit voltage with nanocrystal bandgap in the film. The colour coding corresponds to the colours inFig. 1and the straight line represents a linear fit to the data yielding VOC=0.85 × bandgap/e– 0.42 V. Figure 4: V oc variation with nanocrystal bandgap. Variation of open-circuit voltage with nanocrystal bandgap in the film. The colour coding corresponds to the colours in Fig. 1 and the straight line represents a linear fit to the data yielding V OC =0.85 × bandgap/ e – 0.42 V. Full size image This small driving energy for hole transfer provides a basis for understanding the EQE spectral features that vary across the nanocrystal size series. Although we noted above that photoexcitation of all the various bandgap nanocrystals contributes to the photocurrent (and hence all devices function), this is not the case for photoexcitation of pentacene. The spectra of devices made with the smallest bandgap nanocrystals (0.67–1.06 eV) show a photocurrent contribution from pentacene, evident as a sharp increase in photocurrent on the rising edge of the pentacene absorption near 1.8 eV. In contrast, devices with 1.20 eV nanocrystals do not show a rise at 1.8 eV, and instead show a decrease at the pentacene absorption band due to partial obstruction of light (filtering) that would otherwise excite PbSe. In the intermediate case of devices with 1.08 eV nanocrystals, there are apparent positive pentacene spectral features, but the overall contribution is less than in devices with 1.06 eV nanocrystals. The complete absence of photocurrent from pentacene for the largest gap nanocrystals and hence the absence of photocurrent from singlet excitations is consistent with previous observations on pentacene/C 60 devices [13] . The threshold effect in the EQE spectra for the size series of PbSe devices sets limits on the pentacene state that precedes charge generation. In devices with 0.67–1.06 eV nanocrystals, the presence of the pentacene absorption features in the EQE spectrum indicates that there is net electron transfer from pentacene to nanocrystals. This process is only possible if the excited state in pentacene has sufficient energy to dissociate at the heterojunction. For the ensemble of nanocrystals, there is a distribution of 1S e energies due to both static and dynamic disorder [48] , and the energy relevant to this analysis is the energy of the onset of photocurrent ( E PCO ). We determine the energy of the 1S e state of the nanocrystals, E (1S e ), such that E (1S e )= E (1S h )+ E PCO , where E (1S h ) is the energy of the 1S h nanocrystal state determined from the photoionization onset ( Supplementary Fig. S1 ) and E PCO is the nanocrystal bandgap as above. For devices containing 1.06 eV nanocrystals ( E PCO =0.96 eV), the energy of the 1S h state is −5.1 eV. Taken together, these data suggest that the excitation in pentacene can be ionized at the interface with nanocrystals that have a 1S e state as high as −4.1 eV with respect to vacuum. As a result, we can estimate the lower bound of the excited state that precedes charge separation with PbSe. The UPS data indicate that the difference between the nanocrystal 1S h state and the first ionization feature of pentacene is Δ=0.05±0.05 eV. There is evidently a suitable population of acceptor states to generate significant photocurrent from the device made with 1.06 eV nanocrystals ( E PCO =0.96 eV). To estimate a lower limit on the energy required to ionize the excited state of pentacene, we take the energy difference between the pentacene ionization energy and the energy for the nanocrystal 1S e state. Including systematic error associated with the bandgap onset ( σ sys =+0.06 eV, Supplementary Fig. S5 ), the lower limit for the energy of the pentacene excited state is E pent > E PCO −Δ− σ sys , or E pent >0.85 eV. The analogous results for the device with 1.20 eV nanocrystals, which fail to ionize the excitation on pentacene, can be used to estimate an upper limit on E pent . For 1.20 eV nanocrystals, the bandgap E PCO =1.07 eV, the HOMO-1S h offset Δ=0.07±0.05 eV, and the systematic error σ sys =+0.12 eV. Because the nanocrystal distribution does not have a sufficient fraction of states to act as acceptors for electron transfer from pentacene, the upper limit for the pentacene bound-state energy is E pent < E PCO –Δ, that is, E pent <1.00 eV. We note that excess energy to drive electron transfer would need to be added to the values calculated. However, the small driving energy required for hole transfer (noted above) suggests that the corresponding energy for electron transfer should be insignificant to this analysis. The energy estimates are independent of modelling or specific knowledge about the excited state dynamics of pentacene. However, it is important to note that from photocurrent, photoelectron spectroscopy, and steady-state absorption data, we identify an excited state whose energy is at half the pentacene bandgap (within error). This is the energy expected for the triplet exciton. An alternative possibility is that there is a >0.8 eV energy required to drive electron transfer from pentacene to nanocrystals. However, the transfer of holes evidently requires a negligible driving energy, so this explanation entails an implausible asymmetry between electron and hole transfer. The direct photogeneration of free charge-carriers in pentacene is highly unlikely. As no other long-lived and mobile electronic excitations are expected at this energy, our measurement is thus consistent with photocurrent generation by ionizing triplet excitations from pentacene ( Fig. 5 ). This result provides a direct connection between ultrafast optical studies of singlet fission [11] , [49] , [50] , [51] , [52] and photovoltaic device operation [12] , [29] , [53] . 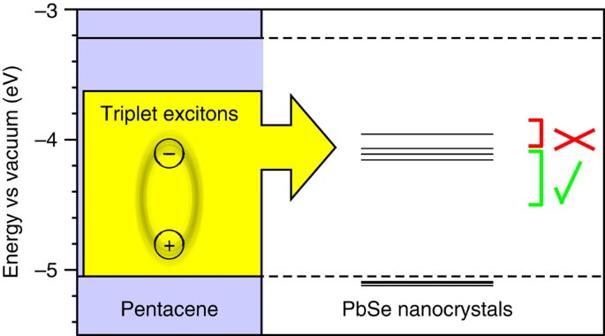Figure 5: Illustration of the threshold for triplet ionization. The dashed lines indicate the HOMO and the LUMO of pentacene films. The solid lines show the position of the nanocrystal bands used in this study. The HOMO of pentacene and the nanocrystal valence-band energies were measured using UPS. The energy levels of nanocrystals with a clear pentacene contribution in the EQE spectra are marked with a tick and the nanocrystals that do not show the full pentacene contribution are marked with a cross. Figure 5: Illustration of the threshold for triplet ionization. The dashed lines indicate the HOMO and the LUMO of pentacene films. The solid lines show the position of the nanocrystal bands used in this study. The HOMO of pentacene and the nanocrystal valence-band energies were measured using UPS. The energy levels of nanocrystals with a clear pentacene contribution in the EQE spectra are marked with a tick and the nanocrystals that do not show the full pentacene contribution are marked with a cross. Full size image Solar cell optimization The correlation between nanocrystal bandgap ( E PCO ) and V oc provides a useful design rule by which to optimize devices. To preserve the advantage of the additional current from pentacene, we design solar cells with E PCO as large as possible while preserving the capability to ionize triplets. Additionally, studies on varying nanocrystal layer thickness showed that our devices performed best for a PbSe layer thickness of 150 nm. We show the EQE and current-voltage characteristic and relevant parameters for the most efficient device (4.7% PCE) in Fig. 6 . The best devices benefit from a small energetic loss between the nanocrystals and pentacene during both hole transfer and triplet ionization, leading to band structures that are well matched. 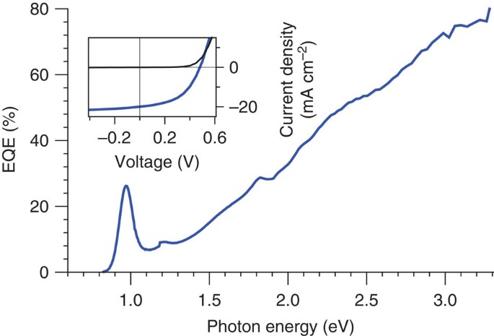Figure 6: Champion device characteristics. EQE and current–voltage characteristics of the best PbSe-pentacene device. The inset shows the current-voltage data, with an open-circuit voltage of 0.48 V, a short-circuit current of 19.9 mA cm−2and a fill factor of 49%, leading to a power conversion efficiency of 4.7% under AM1.5G illumination. The nanocrystal bandgap in the film is 0.98 eV. Figure 6: Champion device characteristics. EQE and current–voltage characteristics of the best PbSe-pentacene device. The inset shows the current-voltage data, with an open-circuit voltage of 0.48 V, a short-circuit current of 19.9 mA cm −2 and a fill factor of 49%, leading to a power conversion efficiency of 4.7% under AM1.5G illumination. The nanocrystal bandgap in the film is 0.98 eV. Full size image Our first devices were relatively unstable under illumination. After continuous illumination for 5 min at 100 mW cm −2 , the devices lost 70% of their initial power-conversion efficiency, although they recovered within minutes of removal from light. This timescale indicates that decreased performance may result from inefficient electron extraction due to interfacial trapping [37] . The evaporation of a 1-nm layer of an electron extraction material, lithium fluoride [54] , between the nanocrystal layer and the aluminium electrode ( Supplementary Fig. S7 ) yielded devices that retained >90% of their performance after continuous illumination. We note that many features of our technique are general, and such a size series can be used to characterize the excited states of other materials. The nanocrystals can transfer holes to any donor material whose HOMO lies above the 1S h energy, and the small driving force required for exciton ionization enables a photocurrent-based analysis for many organic semiconductors [55] . For an appropriate nanocrystal size series, it is also possible to probe the energetic states of organic acceptors through the inverse ionization process [56] . Additionally, the use of alternative materials (for example, CdSe) opens the possibility to probe the states of organic molecules beyond the range accessible by PbSe. The nanocrystal size series thus constitutes an in situ spectrometry for devices, based on quantum-confined materials rather than light. In conclusion, we have fabricated photovoltaic devices with a size series of PbSe nanocrystals and pentacene. Using the nanocrystal size series as a set of electron acceptors with tunable energy, we find that the energy of the pentacene triplet is at least 0.85 eV and at the most 1.00 eV in operating devices. Our solar cells show efficient charge separation and show competitive performance at 4.7% power conversion efficiency with low voltage loss. On the basis of the potential for harvesting multiple excitations with pentacene and on the rapid improvements of singlet-fission sensitized photovoltaics to date, we are optimistic about the use of nanocrystals both as materials to enable high-performance photovoltaic technologies and as tools for basic device characterization. PbSe nanocrystal synthesis We synthesized nanocrystals using modified versions of previously reported methods [36] , [57] . All chemicals were purchased from Sigma Aldrich, if not otherwise stated, and were anhydrous if available. The quantum dot size was controlled by reaction time and injection temperature. For nanocrystals larger than 3 nm (0.6–1.0 eV), Pb(OAc) 2 H 2 O (3.44 mmol; 1.3 g), oleic acid (OA; 8.58 mmol; 2.7 ml) in 1-octadecene (ODE; 75 mmol; 24 ml) were degassed at 70 °C under vacuum (10 −2 mbar or better) for 2 h. To complex lead oleate, the temperature was increased to 160 °C under nitrogen atmosphere. The flask was heated to the desired injection temperature (110–160 °C) and the second precursor solution, containing Se (Alfa Aeser, 10.8 mmol; 852.8 mg) and diphenylphosphine (DPP; 15 μmol; 26.1 μl) in tri- n -octylphosphine (TOP; 24.2 mmol; 10.8 ml), was injected rapidly under nitrogen atmosphere. After 1.5 min to 10 min, the reaction was cooled to 30 °C by placing the flask in room-temperature water. Subsequent purification steps were carried out in a nitrogen-filled glove box. The nanocrystals were extracted via repeated precipitation with a mixture of 1-butanol and methanol. For nanocrystals smaller than 3 nm (1.0–1.3 eV), the procedure is based on a two-fold scale-up of a procedure reported previously [58] . Briefly, lead (II) oxide (16 mmol; 3.56 g) and oleic acid (64 mmol; 20 ml) were dissolved in ODE (10–20 ml, depending on desired nanocrystal size). The solution was degassed at 80 °C at 8×10 −3 mbar (6 mTorr) and then heated over the course of 1 h to 150 °C under nitrogen to form the colourless lead (II) oleate solution. The degassed solution was cooled down to 80 °C. A solution of TOPSe (1.0 mol l −1 , 20 ml) was injected into the lead oleate solution. The reaction temperature was maintained at 80 °C, and after several minutes, the reaction mixture grew dark, signalling the onset of nucleation. Aliquots (diluted with tetrachloroethylene) were used to monitor the progress of growth, which was complete after 15–60 min. We also observed post-growth size focussing in our PbSe samples even after the reaction mixtures have been diluted and cooled to room temperature (similar to reports for PbS [59] ). Nanocrystals were isolated from the reaction mixture by flocculating to turbidity: either using a 1-butanol/methanol/hexanes solvent system (in the case of 1.0 and 1.15 eV bandgap nanocrystals) or an acetone/chloroform solvent system (in the case of the 1.1 and 1.3 eV bandgap nanocrystals). PbSe nanocrystal characterization The absorption spectra of the nanocrystals were taken in solution at 0.05–1 mg ml −1 using a PerkinElmer Lambda 9 UV-Vis-IR spectrophotometer. Optical bandgap, size distribution and size of the nanocrystals have been determined by fitting a Gaussian function to the first excitonic peak in the absorption spectra based on the data provided by Jasieniak et al [44] . UPS/XPS measurements The samples were transferred to the ultrahigh vacuum chamber (ESCALAB 250Xi) for UPS/XPS measurements. UPS measurements were performed using a double-differentially pumped He gas discharge lamp emitting He I radiation ( hν =21.22 eV) with a pass energy of 2 eV. The UPS spectra are shown as a function of binding energy with respect to the vacuum level, and the energy edge of the valence band is used to determine the ionization potential of the measured film [55] . The ionization potential of pentacene was measured to be 5.05 eV, in agreement with previous measurements [45] , [46] . XPS measurements were carried out using a XR6 monochromated X-ray source with a 650-μm spot size. Se 3 d spectra were normalized, so that the intensity of the Pb 4 f spectra represents the stoichiometry of the PbSe nanoparticles. The general trend shows that the smaller nanoparticles are richer in Pb. Device fabrication The devices were fabricated in a sequential bilayer structure. First, a 50-nm thick layer of pentacene was evaporated on top of a pre-patterned ITO slide on glass (Psiotec). Pentacene was evaporated under a vacuum of 2×10 −6 mbar or better at a rate of 0.1 Å s −1 . The samples were kept under nitrogen atmosphere and the nanocrystals were spun in a glovebox (<1 p.p.m. O 2 and H 2 O) in a sequential layer-by-layer technique, following reported methods [60] . The nanocrystals were suspended in octane at 25 mg ml −1 . All solvents and solutions were added directly through a 0.2 μm PTFE filter onto the substrate for spin-coating at 1,500 r.p.m for 10 s after a 3-s wait. A first linker layer was deposited by spin-coating from a 0.02 M (0.23 vol%) solution of 1,3-benzenedithiol in acetonitrile, followed by spin-coating using pure acetonitrile. The same conditions were used to spin the active layer by first depositing a layer of nanocrystals, followed by 1,3-benzenedithiol, acetonitrile and octane. This procedure was repeated until the required thickness was reached. The samples were transferred into a thermal evaporator without removing from the nitrogen atmosphere. Lithium fluoride (1 nm) and aluminium (100 nm) were deposited at 3×10 −6 mbar or better. The devices were encapsulated by attaching a glass slide on top of the contacts using a transparent epoxy. The devices were characterized in air under an Oriel 92250A solar simulator using a Keithley 2636A source measure unit. The incident power was corrected for spectral mismatch in the spectral region from 375 to 1,045 nm. Some of the solar cells absorbed light with wavelengths beyond 1,045 nm; however, even in a worst case scenario, the effect of spectral mismatch does not affect the reported performance by more than 4% for those cells. External quantum efficiency spectra were recorded under monochromatic light from an Oriel Cornerstone 260 monochromator. Error analysis for the triplet energy determination We determine the ionization potential from the UPS data as the onset of the signal (the upper end of the density of states) and the relevant band energy from the onset of EQE signal. Both the method for determining the onset of EQE and of UPS introduce a systematic error as follows. We fit a straight line to the onset of EQE or UPS signal, but the actual shape of the onset of EQE and UPS signal is nonlinear. The error is the difference between the energy of the fit onset and the point at which the signal is discernible from the noise ( Supplementary Fig. S5 ). If the population of nanocrystals that have a bandgap equal to or less than the EQE onset are sufficient to sustain photocurrent in the device (which is what the EQE entails), then this method may overestimate the required energy. The overall systematic error is determined by adding the systematic errors of the UPS and the EQE in quadrature. Statistical error from the fitting process is not quoted for this analysis, as it is nearly two orders of magnitude less than the systematic error. How to cite this article: Ehrler, B. et al . In situ measurement of exciton energy in hybrid singlet-fission solar cells. Nat. Commun. 3:1019 doi: 10.1038/ncomms2012 (2012).